High heat flow and ocean acidification at a nascent rift in the northern Gulf of California The prevailing tectonic setting in the Gulf California suggests the presence of an undetermined number of short spreading centres with associated hydrothermal systems. However, to date, active seafloor spreading phenomena have been documented in only three of the eight tectonically active basins. Here we report heat flow values as high as 15,436 mW m −2 in two of the northernmost basins of the Gulf of California, providing evidence of intense hydrothermal activity associated with the transition from continental rifting to seafloor spreading. The mean heat flow for the Wagner and Consag basins area is 1,875 mW m −2 , more than 15 times higher than the mean value for oceanic crust (105.4 mW m −2 ). Additional evidence for vigorous hydrothermal circulation and a shallow heat source includes intense gas discharge (CO 2 and CH 4 ), widespread low pH (average 7.7), locally high 222 Rn concentrations in the bottom water and a high extent of organic matter maturation in the sediments. The Gulf of California (GC) formed as a result of oblique rifts linked by long transform faults and short spreading centres at ~6 Ma ago [1] . Active seafloor spreading phenomena have been documented in only three of the eight tectonically active basins located in the GC [2] . However, the prevailing tectonic setting in the region indicates that the Gulf likely includes an undetermined number of short spreading centres [3] with hydrothermal systems in different stages of development. The majority of data on active seafloor spreading in the GC corresponds to the Guaymas and the Alarcón basins [4] , [5] . A crustal thickness of ~15 km has been calculated for the northern Gulf [6] , and this area is suited to study the transition from continental to oceanic rifting. The Wagner and Consag basins are located towards the northernmost extent of the GC ( Fig. 1 ) between the Upper Gulf to the north and the Upper and Lower Delfín basins to the south. The two basins are semi-graben structures that link the Upper Delfín basin to the south and the subaerial Cerro Prieto basin to the north in the Mexicali-Imperial Valley along the Pacific–North America plate boundary in the northern GC. These basins are the shallowest basins in the GC, with depths of less than ~225 m, and are tectonically active with a relatively high number of faults [7] . 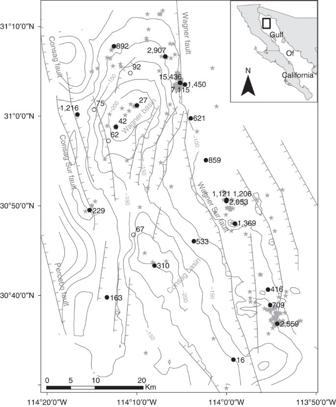Figure 1: Locations of the Wagner and Consag basins and the heat flow stations. Detailed bathymetric map of the Wagner and Consag basins; stars indicate the flare locations. Thick lines denote the main and secondary faults identified by the seismic reflection (Wagner basin faults20; Consag basin faults9). Numbers indicate the heat flow data (values in mW m−2) from this study (filled circles) and previously published results (open circles)3. A majority of values are greater than the mean ocean heat flow18(105.4 mW m−2). Figure 1: Locations of the Wagner and Consag basins and the heat flow stations. Detailed bathymetric map of the Wagner and Consag basins; stars indicate the flare locations. Thick lines denote the main and secondary faults identified by the seismic reflection (Wagner basin faults [20] ; Consag basin faults [9] ). Numbers indicate the heat flow data (values in mW m −2 ) from this study (filled circles) and previously published results (open circles) [3] . A majority of values are greater than the mean ocean heat flow [18] (105.4 mW m −2 ). Full size image Geophysical or geochemical evidence of active seafloor spreading in the northern GC has not been previously reported. Moreover, the Wagner and Consag basins have been considered as unlikely to contain active seafloor spreading processes, despite having the highest density of faults [7] in the northern Gulf as well as possible mantle upwelling under the Wagner basin indicated by seismic modelling [8] . In the Wagner basin, the sediment thickness is greater than 7 km, which impedes the rise of magma generated by seafloor spreading; this hindrance, in turn, masks any visible evidence of rifting [9] . Consequently, heat flow anomalies are the only indication of nascent spreading centres in the sediment-covered basins [10] . The connexion of the two basins to the active spreading centres at Delfin basin and Cerro Prieto has long been hypothesized but not demonstrated [11] , [12] because the thick sediment cover eliminates the possibility of identification of magnetic banding or gravity anomalies related to active ocean spreading. Recently, the occurrence of gas venting has been reported [13] in both of the basins. Beneath the plumes, acoustic blanking is widely observed, indicating subsurface gas accumulation ( Fig. 2a ). Although there are areas on the western side of the basins where surface gas flares are not detected, sub-bottom profiles indicate the disruption of the sedimentary structure by newly ascending gas plumes ( Fig. 2b ), indicating that the activity is increasing. 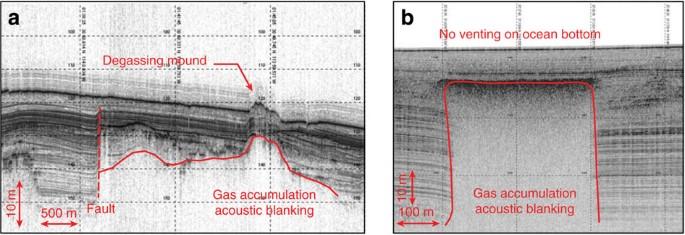Figure 2: Sub-bottom profiles. Sub-bottom profiles showing the blanking effects of gas saturation: (a) zones with active venting in the northeastern region of the study area; (b) new areas of gas upwelling without sea bottom disruption in the western portion of the study area, where a large222Rn anomaly indicates the upflow location (W−27 inSupplementary Fig. S1). Figure 2: Sub-bottom profiles. Sub-bottom profiles showing the blanking effects of gas saturation: ( a ) zones with active venting in the northeastern region of the study area; ( b ) new areas of gas upwelling without sea bottom disruption in the western portion of the study area, where a large 222 Rn anomaly indicates the upflow location (W−27 in Supplementary Fig. S1 ). Full size image Detailed bathymetric mapping of the Wagner and Consag basins ( Fig. 1 ) indicates the eastern edge of the basins bordered by the Wagner Fault. The bathymetry and acoustic sub-bottom profiler data reveal large vertical displacements due to the recent faulting that disrupts the sedimentary column. During two oceanographic cruises, more than 300 flares were mapped on the echo-sounder profiles ( Fig. 1 ) at depths from 65 to 150 m, covering an area of 2,240 km 2 . The gas plumes originate from sites of large disruptions of the upper sediment structure (for example, synsedimentary faults, pockmarks, mud domes and diapirs, as well as raised irregular hard reflectors; Fig. 2a ). The plumes had mainly diffuse and intermittent gas flows in extensive areas of the basins, as observed using a remotely operated vehicle (ROV) camera. The extensive tidal and convective mixing, as well as the strong currents in the Gulf, combine the different water masses, thus maintaining a nearly constant temperature in the bottom of the Wagner and Consag basins [14] , [15] . This effect allows the measurement of the temperature gradient minimizing seasonal variations in the temperature. In contrast, the strong vertical mixing in the water column produces less pronounced physico-chemical profiles related with ocean bottom discharge features [16] . Historical heat flow studies were concentrated in the central and southern part of the GC, and only four heat flow measurements [3] have been performed in the Wagner and Consag basins, producing values in the range from 63 to 92 mW m −2 . Additionally, heat flow values of 108 and 126 mW m −2 near the Wagner and Consag basins were calculated using the Curie point isotherm depths [17] . Previous data did not indicate the presence of a major heat flow anomaly in the northern GC, as the mean heat flow for the oceanic crust [18] is 105.4 mW m −2 . Seismicity is high in this region [9] , [19] , and focal mechanisms are mainly strike-slip and dip-slip, which are consistent with the extension character of the basins and the transform faults of the Cerro Prieto system. The earthquakes recorded between 1973 and 2009 show that significant seismic activity occurs along the main faults on the borders of the basins [9] . The deep structure of the Wagner basin was described based on seismic images that present poor resolution at depth in the Wagner and Consag basins area; however, these data allow for the inference of the basement depth below the 7-km-thick sediment cover [20] . The observed gas accumulation may explain the low quality of the images obtained in the seismic studies. The mapped structures in the upper 4−5 km reveal the presence of abundant faults within both of the basins (1 fault km −1 in Wagner basin and 1.3 faults km −1 in Consag basin [20] ). These faults do not reach the sea bottom ( Fig. 3b ), but they do increase the permeability at depth within the thick sediment pack and allow for convective heat transfer in the deep sedimentary layers. 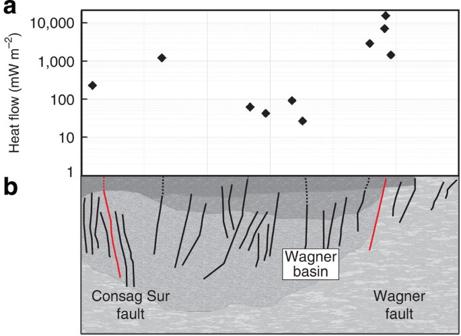Figure 3: Heat flow pattern and faults throughout the Wagner basin. The scheme shows (a) the heat flow variation across the Wagner basin on a SW-NE profile and (b) the main fault location as identified by the seismic reflection data9,20. High values correlate with the presence of the Wagner and Consag Sur faults. Figure 3: Heat flow pattern and faults throughout the Wagner basin. The scheme shows ( a ) the heat flow variation across the Wagner basin on a SW-NE profile and ( b ) the main fault location as identified by the seismic reflection data [9] , [20] . High values correlate with the presence of the Wagner and Consag Sur faults. Full size image The magnetic and gravity anomalies coincide with the centre of the Wagner basin, and their low amplitude is related to the thick sediment cover [17] . A thick sediment cover usually masks lineated anomalies produced by seafloor spreading. Additionally, it has been suggested that the low permeability of the sediments will favour a more intense alteration of any layered intrusions at depth, thereby suppressing the magnetic anomalies [21] . Magnetic surveys indicate that the upper basement in this area likely contains basalt layers interbedded with sediments [17] , [22] . Here, we present new heat flow data and pH measurements, detailed bathymetric observations, gas compositions, profiler sections and organic matter maturation data; this information provides the supporting evidence required to infer the occurrence of active seafloor spreading at the Wagner and Consag basins. The average thermal gradient of ~1 °C m −1 (greater than 30 times the average gradient on Earth) and the occurrence of 222 Rn-positive anomalies in the bottom water samples reveal the occurrence of high heat flow-driven convection through the thick sediment cover, which generates diffuse gas discharge (mainly CO 2 with minor CH 4 ). CO 2 is a common gas discharging from hydrothermal vents, and as CO 2 dissolves in sea water, the pH decreases, thereby generating acidification over an extensive area. The identification of CO 2 as the most abundant gas in the discharged fluids explains the low pH measured in the area and identifies this zone as a natural laboratory to explore the evolution of ecosystems under long-term exposure to low pH conditions. Heat flow measurements In contrast to spreading centres that do not have a sediment cover, the thick sediment layer in the Wagner and Consag basins made it possible to conduct coring and heat flow surveys in the study area, especially over the active hydrothermal manifestations. As this is the first detailed heat flow mapping of the basins, we located the heat flow stations in profiles that crossed the basins to identify heat transport anomalies. We focused the heat flow and coring studies on the trace of the Wagner and Wagner Sur faults, where the majority of the hydrothermal features occur, as this structure likely dominates the deep fluid circulation. The measured thermal gradients varied from 0.01 to greater than 12 °C m −1 (see sample plots in Supplementary Fig. S1 ), and thermal conductivity values were relatively homogeneous with an average of 1.2 W m −1 °C −1 . The calculated heat flow ranged from 16 to 15,436 mW m −2 ( Table 1 , Fig. 1 ). At station 14, the temperatures below 3 m exceed the maximum range of the thermistors (60 °C), and the gradient (>10 °C m −1 ) was calculated using data from only five thermistors, which nevertheless, yielded a good linear correlation ( Supplementary Fig. S1 ). Only three stations presented heat flow values below the mean value for the oceans (105.4 mW m −2 ), and the remaining measurements were well above this value. The calculated error in the heat flow measurements was <10% for all the stations ( Table 1 ) except for station 1 (22.84%), where the lowest heat flow value was obtained. Table 1 Heat flow measurements using the FIELAX probe (11 thermistors*) in the Wagner and Consag basins. Full size table pH and gas chemistry The bottom water samples were collected to determine the pH, dissolved gas concentrations and 222 Rn concentrations. Only CO 2 and CH 4 were detected in the gas sample ([CO 2 ]=78% and [CH 4 ]=22%); in addition, CO 2 was the predominant component of the dissolved gases in bottom water samples collected near flares. The concentration of 222 Rn in the bottom water samples varied within the interval from 0 to 2,430 d.p.m./100 l ( Supplementary Fig. S2 , Supplementary Table S1 ). The data presented here represent the first detailed survey of the seafloor pH in the northern Gulf ( Fig. 4 , Supplementary Table S2 ); previous reports included only one station used to define the pH in the water column in the southern Consag basin [23] . Regional studies that reported pH values at the surface and in the water column along a NW-SE profile of the GC [23] , [24] showed that, in the northern Gulf, the lowest pH value at the surface was 8.29. However, at 200 m depth, all recorded pH values were greater than 7.85 throughout the entire GC. Consequently, the obtained pH values of 7.55–7.85 can be considered as anomalously low and linked to the diffuse flares emitting CO 2 that were found during this study. 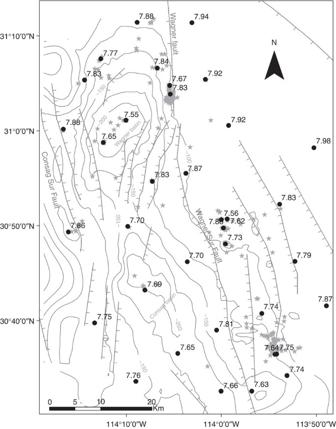Figure 4: pH data of the Wagner and Consag basins. pH values measured in the bottom water samples. A majority of measured values are less than the reported pH for the northern Gulf of California at 200 m depth (7.85)23. Stars indicate the flare locations. Figure 4: pH data of the Wagner and Consag basins. pH values measured in the bottom water samples. A majority of measured values are less than the reported pH for the northern Gulf of California at 200 m depth (7.85) [23] . Stars indicate the flare locations. Full size image Sedimentary organic matter maturation The thick sediment layer present in the Wagner and Consag basins contains abundant organic matter that is altered by the circulating hydrothermal fluids. The ratios between the aliphatic alkanes allowed for the calculation of the proportion of short- to long-chain alkanes (SRL) and the carbon preference index that were used to establish the origin, distribution and maturity level of the sedimentary organic matter (SOM). The carbon preference index values suggest that the high variability in the SOM maturity, which displayed a patchy pattern, was related to the flare occurrence. A similar variability is also observed in the Pr/Ph ratio (pristane/phytane), the presence of polycyclic aromatic hydrocarbons, the pentamethylicosane isoprenoid levels and the elemental ratio between the carbon and hydrogen (C/H) from bitumen. The GC has been experiencing a transition from continental rifting to seafloor spreading since 6 Ma ago [1] . The variations in the rifting style along the Gulf grade from typical seafloor spreading in the southern troughs [2] to continental rifting in the northern end [11] , [12] (Salton Sea, Browley and Cerro Prieto). The northern GC is a typical example of the early stages of this transition. The heat flow in the ocean floor is a key observation for describing seafloor spreading and estimating the energy output related to the associated hydrothermal systems. However, the measured conductive flow is usually lower than that predicted by lithosphere cooling models and is considered unreliable for the estimation of heat flux because in sediment deprived rifts, convective flow dominates heat transfer. However, in sedimented rifts, the low permeability of the sediment layers allows for a dominance of the conductive processes, and heat flow measurements are a good indication of the energy output of the system [25] . In the case of the Wagner and Consag basins, the sediment thickness is 7 km, and the heat discharge estimation can be considered as reliable. Previous heat flow measurements [3] (average 74 mW m −2 ) in the Wagner and Consag basins were located in the deepest areas of the basins, coinciding with the lowest heat flow values that were recorded in this survey ( Fig. 1 ). In contrast, high heat flow is predominant at the basin borders, particularly in the eastern part of the study area at the borders of the Wagner and Wagner Sur faults ( Fig. 3a ), and the highest value was recorded on the northeastern section that was associated with the largest observed flares. The abundance of faults in the Wagner and Consag basins favours convective heat transfer by locally enhancing the sediment permeability. The seismic profiles indicate that most faults extend up to a depth of <500 m and do not reach the sea bottom ( Fig. 3b ). Therefore, shallow sediment layers act as a seal cap, which prevents convective fluid discharge at the sea bottom except for those areas where the major faults intersect the bottom, generate permeable zones in the otherwise impermeable sediments and allow flares to occur. The heat flow pattern throughout the Wagner basin ( Fig. 3a ) differs from the typically observed maximum in the axial depression of the mature seafloor spreading centres [25] . The heat flow value distribution recorded at the Wagner and Consag basins indicates that in their early stages of development, the spreading centres with thick sediment cover present hydrothermal convection that is restricted to the permeable zones defined by active faults; in the shallow sediment layers, heat transport is dominated by conduction. The mean heat flow value of 1,875 mW m −2 corresponds to a calculated thermal output of >4,000 MW th , including only those areas where hydrothermal manifestations have been observed (2,240 km 2 ). This heat output is more than four times the total ‘steady’ hydrothermal heat discharge (~1,050 MW th ) identified in the US part of the Cascade Range [26] . Marine heat flow values of the order of 1,000 mW m −2 have been observed only in areas where active seafloor spreading occurs, such as the Guaymas basin [27] , and values as high as 490,000 mW m −2 have been reported for a sedimented flank at the Juan de Fuca Ridge [28] . High heat flow values and intense seismicity in the Wagner and Consag basins imply the presence of a vigorous hydrothermal system in these basins. The low permeability of the sediment cover, especially in the upper layers, as shown by the sub-bottom profiler images ( Fig. 2a ), produces high conductive heat flow values measured in the ocean bottom as a result of convection in the deeper layers. The measured CO 2 /CH 4 gas ratio of ~4 is consistent with an equilibrium temperature in the order of 200 °C and is typical of sedimentary basins with active hydrothermal systems [29] . High-temperature areas in the Guaymas basin [30] , where thermal stress is evident in the extent of organic matter maturation, are characterized by large amounts of CO 2 and a limited range of hydrocarbons (i.e., predominantly CH 4 ). Therefore, it is likely that the high temperature and thick sediment cover in the Wagner and Consag basins result in the simple composition of the discharged gas (CO 2 and CH 4 ). The predominance of CO 2 in the discharged gas and the extensive occurrence of flares in both of the basins has acidified 20–50 m of sea water near the bottom of the entire area (>2,000 km 2 ) to values within 7.55–7.98 pH T units ( Fig. 4 ; Supplementary Table S2 ). Similar phenomena of extensive sea water acidification generated by CO 2 discharged by hydrothermal venting have not been reported. However, local acidification was observed in three sites [31] , [32] , [33] , namely, the Okinawa Trough, Japan (lowest pH=6.97 at 1,428 m depth), in Ischia, Italy (lowest pH=6.40 at 3 m depth), and in Papua New Guinea (lowest pH=7.21 at 3 m depth). CO 2 venting in those areas is related to the presence of marine deep- and shallow-water hydrothermal systems. The average value of 7.77 units, as found in the present study, is similar to the extrapolated pH level of the shallow ocean water at the end of this century due to the increase in atmospheric CO 2 concentrations [34] . The extensive acidification of the bottom water predominates over the mixing effect of strong currents and makes this area a natural laboratory for the study of the effects of long-term acidification on deep-water ecosystems. The water column radon anomalies in the basins indicate the input of excess radon due to injection from a 222 Rn-rich fluid. The maximum observed 222 Rn value of 2,430 d.p.m./100 l is well above the 60 d.p.m./100 l level that was measured in bottom water samples from the Juan de Fuca ridge flank [28] , which is an area with intense hydrothermal circulation and a thermal output of 1.5 MW. The positive anomalies of 222 Rn along the Wagner Fault coincide with the presence of the strongest flares, suggesting hydrothermal circulation in the thick sediment cover and revealing the location of upflow areas. High values were also observed in the areas with incipient upflow, as shown in Fig. 2b and Supplementary Fig. S1 . Further evidence of the presence of hydrothermal activity in the Wagner and Consag basins is provided by the SOM alteration. Maturation of SOM due to intense hydrothermal activity in heavily sedimented rifts generates plumes of low molecular weight hydrocarbons [35] . The highest maturity values correlate well with the observed presence of the flares. Furthermore, the identification of the pentamethylicosane isoprenoid, related to Crenarchaeota [36] that live at temperatures between 75 and 105 °C, is important evidence of the occurrence of hydrothermal activity; this compound has been associated with methanogenic bacteria [37] , and its presence coincides with the location of the largest flares in the northeastern Wagner basin. The data reveal that hydrothermal circulation occurs along the main structures, especially the Wagner and Wagner Sur faults, and that the anomalously high heat flow values support the association with active seafloor spreading and mantle upwelling in the Wagner and Consag basins. Both basins display all of the typical characteristics of sediment-covered active oceanic ridges with a large heat flux. However, in this case, the large heat flow values are restricted to the higher-permeability areas related to the trace of the largest faults, indicating that the transition from ‘continental rift to seafloor spreading’ remains in the early stages with the presence of asymmetrical semi-grabens and no geophysical evidence of oceanic lithosphere formation. However, the average heat flow agrees well with the calculated values for the conductive cooling of very young lithosphere. This characterization demonstrates that the continental rifting to the seafloor spreading transition is highly advanced in the GC and extends to the northernmost area. Bathymetry and acoustic sediment profiler The data presented here were collected during two oceanographic cruises, WAG-01 (2007) and WAG-02 (2010), aboard the R/V El Puma. The survey tracks were ~4,500 km in length and covered an area of ~3,500 km 2 (~90 km × 40 km), which included the Wagner and Consag basins. The survey paths for the second cruise were planned based on the location of the active flares to cover those areas with additional detailed bathymetry and sampling stations. Three types of Kongsberg echosounders were used: an 18 kHz Simrad ES-60 and a 120 kHz Simrad EY-60 and Multi Beam EM300. The bathymetry data were processed using the Fledermouse software. A Kongsberg TOPAS parametric acoustic sub-bottom profiler (used in Chirp mode from 1 to 6 kHz) with a sub-seafloor penetration of several tens of metres was used to study sediment features and structures, including blanking due to gas saturation. The data were displayed using the Kongsberg TOPAS software. Autonomous underwater vehicle missions In four sites, we used the ROV SeaEye LINX to observe the gas vents and take bottom water samples. Water and gas chemistry The bottom water samples were collected using standard Niskin bottles attached to the ROV. Samples from ~10 m from the ocean bottom were collected using a Rosette Water Sampling System, and samples from ~1 m above the seafloor were obtained using hydrocasts. The gas analyses were performed on board the ship using two packed-column gas chromatography (GC) systems with thermal conductivity and flame ionization detection. The interstitial gas in vials was analysed in the laboratory using gas chromatography mass spectrometry (GC–MS; Polaris Q). The sea water samples for 222 Rn measurements were collected near the seafloor and taken directly from the Niskin bottles while avoiding contact with air using special glass containers of 250 ml. The containers were connected to an Electronic Radon Detector ‘RAD 7’ coupled with an additional ‘RAD-H 2 O’ radon-in-water accessory (Durridge Co.) to measure the 222 Rn concentrations in the sea water samples. On board the ship, the water subsamples were collected in glass bottles, and the pH T (in total scale) was immediately measured using a pH meter with an accuracy of 0.01 pH units. The total alkalinity ( A T ) was measured by Gran titration. The parameters of the carbonate system ( p CO 2 , CO 3 2− , HCO 3 − , C T and saturation state of calcite (Ω c ) and aragonite (Ω a )) were calculated based on the pH T , mean A T , temperature and salinity at the sampling depth pressure using the free-access CO 2 SYS package [38] . A T was nearly constant at all sites; therefore, its mean was used to calculate the carbonate chemistry parameters ( A T =2,359.01 μmol kg −1 ). The mean values of pH T were calculated from hydrogen ion concentrations and then converted back to pH values [39] (available at http://cdiac.ornl.gov/oceans/co2rprt.html ). Organic matter maturation in sediments The sediment sampling was performed using a Smith–McIntyre grab sampler, a USNEL box corer and a gravity corer. The sediment samples used in the organic matter analysis were maintained frozen until they were brought to the laboratory. Subsequently, the soluble organic matter was extracted and analysed by gas chromatography (Gas Chromatograph 5973 Network, injector 7683 B, coupled to MS Hewlett-Packard Agilent 6890N). Heat flow measurements Heat flow measurements were performed using a 6-m-long FIELAX probe with 11 thermistors. The full length of the probe penetrated the sediment during all of the measurements, and the ocean bottom temperature was recorded. The data were processed using custom software based on the codes published by Villinger and Davis [40] . The high sedimentation rate (3.77 cm year −1 ) [41] decreases the measured heat flow values. The data were not corrected for sedimentation, and thus, the presented heat flow data should be taken as the minimum possible values because the actual values would be much higher. Seasonal changes in the bottom temperature were not significant due to strong mixing phenomena [14] . How to cite this article: Prol-Ledesma, R.M. et al. High heat flow and ocean acidification at a nascent rift in the northern Gulf of California. Nat. Commun. 4:1388 doi: 10.1038/ncomms2390 (2012).